A sub-nanometre view of how membrane curvature and composition modulate lipid packing and protein recruitment Two parameters of biological membranes, curvature and lipid composition, direct the recruitment of many peripheral proteins to cellular organelles. Although these traits are often studied independently, it is their combination that generates the unique interfacial properties of cellular membranes. Here, we use a combination of in vivo , in vitro and in silico approaches to provide a comprehensive map of how these parameters modulate membrane adhesive properties. The correlation between the membrane partitioning of model amphipathic helices and the distribution of lipid-packing defects in membranes of different shape and composition explains how macroscopic membrane properties modulate protein recruitment by changing the molecular topography of the membrane interfacial region. Furthermore, our results suggest that the range of conditions that can be obtained in a cellular context is remarkably large because lipid composition and curvature have, under most circumstances, cumulative effects. Cellular organelles display large differences in lipid composition [1] , [2] . At one extreme, the endoplasmic reticulum (ER) is characterized by the abundance of lipids with monounsaturated acyl chains, the scarcity of negatively charged phospholipids and low levels of cholesterol ( ca . 5 mol%). At the other extreme, the plasma membrane (PM) contains high levels of saturated lipids, of cholesterol (up to 30 mol%) and of negatively charged phospholipids, which concentrate in the cytosolic leaflet. As a result of these differences, transmembrane proteins travelling along the ER—Golgi—PM route and peripheral proteins transiently associating with these organelles experience different lipid environments [3] , [4] , [5] . For example, membrane electrostatics provided by negatively charged lipids directs the attachment of many proteins underneath the PM. More obscure is the role of phospholipid unsaturation: why, through complex acylation–deacylation reactions, does the cell need to change the fatty acid profile of its most abundant phospholipids after their synthesis in the ER [6] , [7] ? Straight saturated acyl chains, together with cholesterol, pack tightly and contribute to the function of the PM as a cell-protecting barrier by reducing its permeability [1] . On the other hand, phospholipids with ‘kinked’ monounsaturated acyl chains (for example, oleate, C18:1) are less prone to align than saturated ones, especially at low cholesterol levels. Consequently, membranes rich in monounsaturated lipids, notably the ER and cis -Golgi, should contain defects in the geometrical arrangement of their lipids. A second factor that should accentuate lipid-packing defects in membranes of the early secretory pathway is curvature. A large fraction of the ER consists of thin (radius 30 nm) tubules, and traffic pathways between the ER and the cis -Golgi also involve the formation of small transport vesicles (radius 30 nm) [8] . Curving a lipid membrane necessarily induces the tilting of its lipids, an effect that should favour exposure of hydrophobic cavities. Overall, lipid-packing defects might be advantageous for several functions of early secretory organelles and notably for their biosynthetic functions [5] . Thus, loose lipid packing at the ER has been suggested to favour the folding of nascent transmembrane proteins. Indeed, when the levels of cholesterol and/or saturated phospholipid accidently increase, this promotes a stress characterized by the accumulation of unfolded transmembrane proteins. In turn, this stress triggers a response characterized by the upregulation of a fatty acid desaturase (Ole1 in yeast) and the arrest of cholesterol synthesis [9] , [10] , [11] , [12] . In addition, several peripheral proteins involved in various functions (lipid transfer, autophagy, nuclear pore formation, vesicle tethering and protein coat dynamics) seem to recognize lipid-packing defects by adsorbing preferentially to positively curved membranes through the insertion of long amphipathic sequences [4] , [13] , [14] , [15] , [16] , [17] . However, lipid-packing defects remain an elusive concept owing to the difficulty in performing structural studies on membranes [18] . Most lipids are flexible molecules and, through shape adjustment, might minimize unfavourable exposure of their hydrocarbon chains to water. In addition, lipids with non-cylindrical shape (for example, lysolipids or diacylglycerols) could distribute non-randomly within regions of different curvature to reduce geometrical mismatches, although the efficiency of such a mechanism has been questioned due to the propensity of lipids to readily mix through the entropic effect [19] , [20] , [21] , [22] , [23] , [24] . In this study, we provide a first comprehensive map of the distribution of lipid-packing defects in model membranes of various shape and composition. For this, we combine coarse grain (CG) molecular dynamics (MD) simulations and a new topographical analysis of the bilayer surface [25] , [26] . We validate the relevance of this in silico approach by showing that the binding properties of a model peripheral protein that is hypersensitive to lipid shape and membrane curvature correlate with the distribution of lipid-packing defects as assessed by simulations. Our study (i) provides the first quantitative description of a crucial but poorly characterized property of cellular membranes, (ii) indicates that lipid-packing defects are intimately related to the concept of membrane bending energy used in continuum physics and (iii) demonstrates that lipid composition and membrane curvature synergize rather than oppose in the formation of lipid-packing defects. This last point explains the binding properties of some membrane curvature sensors and is of crucial importance in chemical biology considering that many natural and synthetic compounds have to partition at the surface of lipid membranes to reach their targets. Effect of lipid unsaturation on ArfGAP1 localization Our model protein for the detection of lipid-packing defects is ArfGAP1, a protein that controls the lifetime of the small G protein Arf1 at the Golgi apparatus. Numerous in vitro studies suggest that ArfGAP1 recognizes membrane curvature through the adsorption of two amphipathic lipid-packing sensor motifs (ALPS) [13] , [14] , [15] , [27] . ALPS are short amphipathic helices that display a peculiar chemistry: their polar face is scarce in charged residues and abundant in serines and threonines, while their hydrophobic face mostly contains bulky hydrophobic residues. ALPS motifs fold at the surface of artificial liposomes displaying high curvature (radius<50 nm) or containing conical lipids (for example, C18:1-C18:1-phospholipids); hence, the idea that bulky hydrophobic residues of ALPS motifs recognize lipid-packing defects that arise from membrane curvature and/or from ‘kinks’ in monounsaturated acyl chains. Recently, Gcs1p, the yeast homologue of ArfGAP1, has been shown to lose its Golgi localization when yeast cells accumulate phospholipids with saturated acyl chains [10] , suggesting that the detection of lipid-packing defects by ALPS motifs occurs in a cellular context. To determine whether this behaviour is conserved in mammalian cells, we expressed enhanced green fluorescent protein (EGFP)-ArfGAP1 in immortalized retinal pigmental cells (RPE1) and determined its localization by fluorescent microscopy after feeding the cells with a saturated (C16:0, palmitate) or with a monounsaturated (C18:1, oleate) fatty acid. Palmitate and oleate predominate in biological membranes and their relative abundance should dictate the formation of lipid-packing defects. To prevent interferences with Arf1-dependent mechanisms and make EGFP-ArfGAP1 a sole reporter of lipid-packing defects, the protein was rendered catalytically inactive by the R50K mutation. Quantitative analysis of cellular phospholipids by gas chromatography revealed that the fatty acid profile of RPE1 cell phospholipids varied accordingly to the imposed diet, showing a two-fold increase in the C18:1/C16:0 ratio with exogenously added C18:1 compared with C16:0 ( Fig. 1a ). Under the same conditions, we observed by fluorescence microscopy that the Golgi/cytosol ratio of ArfGAP1 increased by two-fold ( Fig. 1b and Supplementary Fig. 1 ). As a control, we determined the localization of ArfGAP3, a functional homologue of ArfGAP1. ArfGAP3 does not contain any ALPS motif and is mostly regulated by interactions with the COPI coat instead of protein–lipid interactions [28] , [29] . In contrast to ArfGAP1, ArfGAP3 was not affected by fatty acid treatments (compare Fig. 1b,c ). Last and to better quantify the effect of lipid unsaturation on ArfGAP1 localization, we prepared a cell line stably expressing EGFP-ArfGAP1(R50K). With these cells, rounds of ArfGAP1 association with the Golgi could be observed by alternating the diet between C16:0 and C18:1 fatty acids ( Fig. 1d ). These experiments indicate that ArfGAP1 is sensitive to phospholipid unsaturation in vivo. 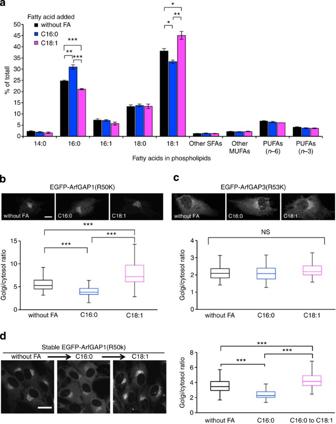Figure 1: Effect of saturated (C16:0) and mono-unsaturated (C18:1) fatty acids (FA) on the localization of ArfGAP proteins. (a) Fatty acid profile of the total phospholipid pool of RPE1 cells after 3 h incubation in the presence of non-lipidated BSA (25 μM) or the indicated BSA–fatty acid complex (25 μM BSA+125 μM fatty acid). Data shown are mean±s.e.m. fromn=4 independent experiments and were analysed by a Bonferroni test after analysis of variance. *P<0.05; **P<0.01; ***P<0.001. (b) Transient expression of EGFP-ArfGAP1(R50K) in RPE1 cells. The starved cells were treated with or without BSA–fatty acid complexes and then fixed. The fluorescence intensity of the protein in the Golgi and in the cytosol was then quantified. (c) Same as inbwith EGFP-ArfGAP3(R53K). (d) RPE1 cells stably expressing EGFP-ArfGAP1(R50K) were submitted to alternating 3-h diets with C16:0 or C18:1 fatty acids in complex with BSA. The cells were imaged over time and the localization of EGFP-ArfGAP1(R50K) was quantified. The box-and-whisker plots inb–dwere built fromn=3 independent experiments (seeSupplementary Fig. 1for all raw data) and show the median (horizontal bar), first and third quartiles (box) and range (vertical bar) of all values. Data were analysed by Kruskal–Wallis and two-tailed Mann–WhitneyU-tests with Bonferroni correction; ***P<0.001; NS, not significant. Scale bar, 10 μm (b); 20 μm (d). SFA: saturated fatty acid; MUFA: mono-unsaturated fatty acid; PUFA: poly-unsaturated fatty acid. Figure 1: Effect of saturated (C16:0) and mono-unsaturated (C18:1) fatty acids (FA) on the localization of ArfGAP proteins. ( a ) Fatty acid profile of the total phospholipid pool of RPE1 cells after 3 h incubation in the presence of non-lipidated BSA (25 μM) or the indicated BSA–fatty acid complex (25 μM BSA+125 μM fatty acid). Data shown are mean±s.e.m. from n =4 independent experiments and were analysed by a Bonferroni test after analysis of variance. * P <0.05; ** P <0.01; *** P <0.001. ( b ) Transient expression of EGFP-ArfGAP1(R50K) in RPE1 cells. The starved cells were treated with or without BSA–fatty acid complexes and then fixed. The fluorescence intensity of the protein in the Golgi and in the cytosol was then quantified. ( c ) Same as in b with EGFP-ArfGAP3(R53K). ( d ) RPE1 cells stably expressing EGFP-ArfGAP1(R50K) were submitted to alternating 3-h diets with C16:0 or C18:1 fatty acids in complex with BSA. The cells were imaged over time and the localization of EGFP-ArfGAP1(R50K) was quantified. The box-and-whisker plots in b – d were built from n =3 independent experiments (see Supplementary Fig. 1 for all raw data) and show the median (horizontal bar), first and third quartiles (box) and range (vertical bar) of all values. Data were analysed by Kruskal–Wallis and two-tailed Mann–Whitney U -tests with Bonferroni correction; *** P <0.001; NS, not significant. Scale bar, 10 μm ( b ); 20 μm ( d ). SFA: saturated fatty acid; MUFA: mono-unsaturated fatty acid; PUFA: poly-unsaturated fatty acid. Full size image Sub-nanometre description of lipid-packing defects To investigate whether the observed cellular behaviour could be attributed to specific changes in membrane microscopic properties, we turned to an in silico approach based on CG MD simulations able to model planar and curved lipid assemblies while retaining chemical specificity [30] . The all-atom (AA) and CG models of the lipids used in this study are shown in Fig. 2a . 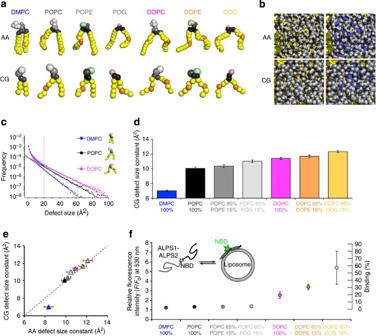Figure 2: Identification of lipid-packing defects in AA and CG MD simulations and correlation with the membrane partitioning of an ALPS peptide. (a) AA and CG VdW representations of the lipid species modelled in this study. Acyl chain carbons involved in single bonds: yellow; acyl chain carbons involved in double bonds: orange; glycerol: black; phosphate: dark grey, choline: light grey; ethanolamine; green; hydroxyl: pink. (b) Top view of POPC bilayers in AA (upper panels) and CG (lower panels) MD simulations. In the right panels, lipid-packing defects, that is, cavities of depth >1 Å below the glycerol (blue) are identified by scanning the membrane surface with vertical lines. (c) Plots of lipid-packing defect frequency versus lipid-packing defect size as determined from thousands of CG MD snapshots for DMPC (blue), POPC (black) and DOPC (magenta) bilayers. Straight lines are linear regression fits forx>20 Å2. (d) Defect size constants as determined from linear fits similar tocin CG simulations of bilayers of different compositions. (e) Correlation between defect size constants in CG and AA flat bilayers for the lipid compositions shown ind. (f) Membrane partitioning of NBD-labelled ALPS1-ALPS2 in the presence of large liposomes (extruded with a 0.4-mm filter, resulting radii >140 nm) of the same lipid compositions as those studied by MD. The plot shows the fluorescence increase of the NBD probe (measured at 530 nm) normalized to the level in solution (F/F0) arising from binding of ALPS1-ALPS2 to the liposome surface. The right vertical bar reports the % of binding as calculated from (F−F0)/(Fmax−F0) (seeSupplementary Fig. 2). Data shown infindicate mean±range from two independent experiments (DMPC, POPC, POPC/POPE and POPC/POG) and from four independent experiments (DOPC, DOPC/DOPE and DOPC/DOG). Error bars ind,eindicate s.e. of regression coefficient estimated during the fitting procedure. Figure 2: Identification of lipid-packing defects in AA and CG MD simulations and correlation with the membrane partitioning of an ALPS peptide. ( a ) AA and CG VdW representations of the lipid species modelled in this study. Acyl chain carbons involved in single bonds: yellow; acyl chain carbons involved in double bonds: orange; glycerol: black; phosphate: dark grey, choline: light grey; ethanolamine; green; hydroxyl: pink. ( b ) Top view of POPC bilayers in AA (upper panels) and CG (lower panels) MD simulations. In the right panels, lipid-packing defects, that is, cavities of depth >1 Å below the glycerol (blue) are identified by scanning the membrane surface with vertical lines. ( c ) Plots of lipid-packing defect frequency versus lipid-packing defect size as determined from thousands of CG MD snapshots for DMPC (blue), POPC (black) and DOPC (magenta) bilayers. Straight lines are linear regression fits for x >20 Å 2 . ( d ) Defect size constants as determined from linear fits similar to c in CG simulations of bilayers of different compositions. ( e ) Correlation between defect size constants in CG and AA flat bilayers for the lipid compositions shown in d . ( f ) Membrane partitioning of NBD-labelled ALPS1-ALPS2 in the presence of large liposomes (extruded with a 0.4-mm filter, resulting radii >140 nm) of the same lipid compositions as those studied by MD. The plot shows the fluorescence increase of the NBD probe (measured at 530 nm) normalized to the level in solution ( F / F 0 ) arising from binding of ALPS1-ALPS2 to the liposome surface. The right vertical bar reports the % of binding as calculated from ( F − F 0 )/( F max − F 0 ) (see Supplementary Fig. 2 ). Data shown in f indicate mean±range from two independent experiments (DMPC, POPC, POPC/POPE and POPC/POG) and from four independent experiments (DOPC, DOPC/DOPE and DOPC/DOG). Error bars in d , e indicate s.e. of regression coefficient estimated during the fitting procedure. Full size image Among all possible membrane parameters, we focused on interfacial lipid-packing defects, as (i) this concept has been put forward to rationalize the observation that curvature and lipid composition influence the adsorption of peripheral proteins to lipid bilayers and (ii) atomistic simulations have shown that ALPS motifs partition into lipid bilayers by inserting their hydrophobic residues into pre-existing hydrophobic cavities [15] . Specifically, all simulations were analysed using a new method aimed at giving a topographic view of the lipid membrane surface [26] . In brief, we identified interfacial lipid-packing defects by discretizing the bilayer with a cartesian grid of 1-Å resolution and by scanning the normal to the membrane plane up to 1 Å below the average level of the glycerol moieties of the lipids [26] ( Fig. 2b ). Lipid-packing defects were identified as regions where no Van der Waals (VdW) lipid density was encountered. As lipid-packing defects are an intrinsically atomic-scale phenomenon, we assessed the ability of CG force fields to provide a reliable description of this property as compared with AA-MD simulations. To analyse the effect of fatty acid saturation, we changed the number of monounsaturated acyl chain in phosphatidylcholine (PC) using the series dimyristoyl-phosphatidylcholine (DMPC) (C14:0-C14:0), palmitoyl-oleoyl-phosphatidylcholine (POPC) (C16:0-C18:1) and dioleoyl-phosphatidylcholine (DOPC) (C18:1-C18:1). Conversely, and to analyse the effect of polar head size, we replaced some PC molecules by phosphatidylethanolamine (PE) (palmitoyl-oleoyl-phosphatidylethanolamine (POPE) or dioleoyl-phosphatidylethanolamine (DOPE)) or diacylglycerol (palmitoyl-oleoyl-glycerol (POG) or dioleoylglycerol (DOG)) giving the following binary mixtures: POPC/POPE, POPC/POG, DOPC/DOPE and DOPC/DOG bilayers at a 85:15 molar ratio. For all compositions studied, plotting the occurrence of interfacial packing defects versus their size shows a single exponential distribution for values>20 Å 2 ( Fig. 2c ; only three representative compositions are shown for clarity). Interestingly, this value is comparable to the minimum defect size required for the insertion of small (alanine and valine) hydrophobic residues in atomistic simulations [15] and to the VdW cross-section of the CG beads used in this study [31] , that is, the resolution of the simulations. As an analogous single exponential behaviour was observed in atomistic simulations [25] , [26] , it is possible to use the defect size constant, that is, the inverse of the exponential decay constant ( Fig. 2c ), as a univocal parameter to quantify interfacial packing defects in lipid bilayers. As shown in Fig. 2d , the CG simulations predict that increasing the number of monounsaturated acyl chains (that is, C18:1 at the expense of C16:0 or C14:0) or introducing lipids with smaller polar heads (for example, diacylglycerol or PE at the expense of PC) are two effective strategies to increase packing defects in flat lipid bilayers, with the defect size constant increasing from 7.0 Å 2 for a pure DMPC bilayer to 12.3 Å 2 for a DOPC/DOG(85:15) bilayer. Even though the AA to CG mapping is not homogeneous for all lipids tested (for example, the replacement of four heavy atoms by one CG bead is not straightforward for the polar head of diacylglycerol and for the acyl chains of DMPC), the quantitative agreement between the defect size constants computed using CG or AA force fields is truly remarkable ( Fig. 2e ). To experimentally validate these results, we assessed the membrane partitioning of an ALPS-containing peptide using liposomes of the same composition as that used in the simulations ( Fig. 2f and Supplementary Figs 2 and 3 ). The ALPS1-ALPS2 motif peptide of ArfGAP1 was covalently labelled with the environment-sensitive probe NBD (N,N′-dimethyl-N-(iodoacetyl)-N′-(7-nitrobenz-2-oxa-1,3-diazol-4-yl)ethylenediamine) and the increase in NBD fluorescence was used as an index of ALPS1-ALPS2 binding to large unilamellar vesicles [14] , [27] (see also Supplementary Figs 2 and 3 ). As shown in Fig. 2f , the fluorescence intensities follow the same order as the defect size constants observed in the CG simulations ( Fig. 2d ). Thus, above a specific threshold, the partitioning of ALPS1-ALPS2 increases strongly with the number of unsaturated acyl chains (DOPC>POPC). Reducing the polar head size while keeping the acyl chains constant also favours peptide partitioning (DOPC/DOG>DOPC/DOPE>DOPC). The comparison between the binding experiments ( Fig. 2f ) and the packing defects computed in the MD simulations ( Fig. 2d ) suggests that the peptide starts binding to lipid bilayers when the defect size constant is above 11.0 Å 2 (for POPC/POG bilayers). This threshold probably reflects the microscopic interactions that a specific protein must engage with the membrane to adsorb efficiently and its knowledge will be crucial to compare several lipid compositions and membrane curvatures. In line with this hypothesis, we observed that two other ALPS motif-containing sequences showed a similar sensitivity to lipid composition as ALPS1-ALPS2 but with a higher threshold value for the defect size constant (12 Å 2 instead of 11 Å 2 , Supplementary Fig. 3 ). Correlation between continuous and atomic models Next, we addressed the role of curvature in the modulation of lipid-packing defects. Curving a membrane is believed to generate a lateral stress that alters the compact arrangement of the lipids in the bilayer, ultimately leading to the formation of lipid-packing defects that are sensed by peripheral proteins [32] , [33] , [34] , [35] , [36] , [37] . This sensing behaviour is illustrated in Fig. 3a , where NBD-labelled ALPS1-ALPS2 was incubated with POPC liposomes of various radii. In agreement with previous observations [13] , [14] , [27] , [38] , membrane partitioning of this motif depended acutely on membrane curvature, with almost no binding on large ( R >100 nm; curvature<0.02 nm −1 ) liposomes and complete binding on small ( R =25 nm; curvature=0.08 nm −1 ) liposomes. The curvature threshold for the binding of the ALPS1-ALPS2 tandem was lower than that observed for simple ALPS motifs (0.02 and 0.05–0.06 nm −1 , respectively; Supplementary Fig. 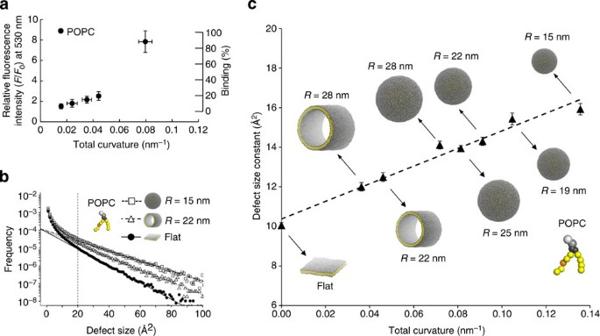Figure 3: Contribution of curvature to the formation of lipid-packing defects. (a) NBD-labelled ALPS1-ALPS2 motif was incubated with POPC liposomes of defined size and its membrane partitioning was determined by measuring the relative NBD fluorescence at 530 nm normalized to the fluorescence of the soluble protein. (b) Occurrence of packing defects versus defect size in the outer leaflet of POPC bilayers from CG simulations of vesicles and tubules of defined curvature. A linear regression fit forx>20 Å allows determining the defect size constant. (c) Defect size constant in the outer leaflet of POPC bilayers as a function of total curvature. The defect size constant was determined from distribution plots similar to those shown inb. Note the linear relationship between the packing-defect size constant and the total membrane curvature. Data shown inaindicate mean±s.d. from three independent experiments. Error bars incindicate s.e. of regression coefficient estimated during the fitting procedure. 4 ) Figure 3: Contribution of curvature to the formation of lipid-packing defects. ( a ) NBD-labelled ALPS1-ALPS2 motif was incubated with POPC liposomes of defined size and its membrane partitioning was determined by measuring the relative NBD fluorescence at 530 nm normalized to the fluorescence of the soluble protein. ( b ) Occurrence of packing defects versus defect size in the outer leaflet of POPC bilayers from CG simulations of vesicles and tubules of defined curvature. A linear regression fit for x >20 Å allows determining the defect size constant. ( c ) Defect size constant in the outer leaflet of POPC bilayers as a function of total curvature. The defect size constant was determined from distribution plots similar to those shown in b . Note the linear relationship between the packing-defect size constant and the total membrane curvature. Data shown in a indicate mean±s.d. from three independent experiments. Error bars in c indicate s.e. of regression coefficient estimated during the fitting procedure. Full size image Considering that the physiologically relevant range of curvatures (defined as J=c 1 +c 2 , where c 1 =1/R 1 and c 2 =1/R 2 are the inverse of the principle curvature radii) lies between J= 0 nm −1 (flat geometry) and J= 0.1 nm −1 (for example, cellular vesicles of R ≈20 nm) [8] , we generated in silico POPC lipid vesicles and tubules of radii ranging from 15 to 28 nm through spontaneous self-assembly of lipid–water mixtures. Thereafter, lipids were allowed to equilibrate between the inner and outer leaflets [39] , [40] ( Supplementary Fig. 5 ) and the packing defects were computed by using a scanning method similar to that used on flat membranes, except that spherical or cylindrical coordinates were used to map the curved bilayer surface (see Methods and Supplementary Fig. 6 ). Figure 3b shows that the occurrence of packing defects versus size remains single exponential even at small curvature radii, thus indicating that the defect size constant is a good parameter to compare flat and curved bilayers. Snapshots of the various simulations are shown in Fig. 3c to illustrate the relative curvature of these model membranes. As expected, lipid-packing defects in the external leaflet of a curved bilayer increase with total curvature ( Fig. 3c ), with the defect size constant ranging from 10.0 Å 2 in flat POPC bilayers to 13.9 Å 2 for R =25 nm POPC vesicles and up to 15.9 Å 2 for R =15 nm POPC vesicles. The observed increase in packing defects is coupled to both an increase in area per lipid ( Supplementary Table 1 ) and an increase in acyl chain ordering in the outer leaflet [40] , in analogy with what is observed in flat bilayers with a high content of conical lipids [26] . Importantly, the computed defect size constant varies linearly with total curvature ( Fig. 3c ), suggesting that the distribution of lipid-packing defects of a membrane can be interpreted as the translation in molecular terms of a macroscopic parameter, curvature, used in physics to describe membrane elasticity [8] , [24] , [41] . Another implication of the linear relationship between the defect size constant and membrane curvature is that fitting the values with a linear regression should give a good estimate of the variations in lipid packing as a function of curvature (caution must be used when extending this analysis to small, non-physiological and fusion-prone vesicles). This implies that at least for constant lipid compositions, only a few points are necessary to compute the response of lipid-packing defects as a function of curvature. As a corollary and because Golgi vesicles, ER vesicles and ER tubules have similar radii (≈25–30 nm), proteins that are sensitive to lipid packing should bind more favourably to vesicles than to tubules, assuming roughly similar lipid compositions. Cumulative effects of lipid shape and membrane curvature Both lipid composition and curvature concur to modulate the number and size of lipid-packing defects in model membranes. However, in a cellular context, it is their combination that gives rise to the unique interfacial properties of membranes [4] . To understand how membrane interfacial properties vary simultaneously as a function of curvature and lipid composition, we first analysed the effect of curvature for bilayers containing phospholipids with different number of monounsaturated acyl chains. To this end, we compared DMPC, POPC and DOPC bilayers in a series that included flat lipid bilayers, a tubule of radius R =22 nm, and two vesicles of radii R =28 nm and R =15 nm, respectively. The defect size constants of these various model lipid membranes were plotted as a function of the total membrane curvature ( Fig. 4a ). 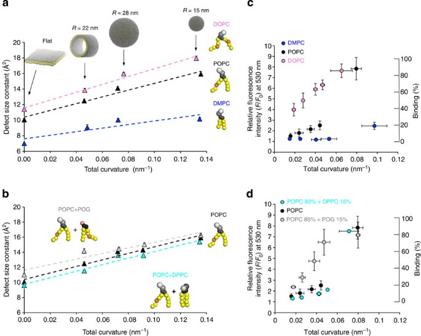Figure 4: Relative contribution of curvature and lipid composition to the formation of lipid-packing defects. (a) Packing defect size constants in the outer leaflet of DMPC (blue), POPC (black) and DOPC (magenta) lipid bilayers as a function of total curvature. Linear regression fits are also shown. (b) Outer leaflet packing defect size constants in POPC (black), POPC/POG (molar ratio: 85:15, light grey) and POPC/DPPC (molar ratio: 85:15, cyan) bilayers as a function of total curvature. Linear regression fits are also shown. (c,d) Curvature-dependent membrane partitioning of ALPS1-ALPS2 in the presence of liposomes of the same compositions as those simulated ina,b. Error bars ina,bindicate s.e. of regression coefficient estimated during the fitting procedure. Vertical error bars inc,dindicate the variation in the relative fluorescence intensity at 530 nm (normalized with respect to the fluorescence of the soluble protein) in two (DMPC, DOPC, POPC/DPPC) or three (POPC, POPC/POG) independent experiments. The horizontal error bars indicate the variation in liposome radius as assessed by dynamic light scattering. Figure 4: Relative contribution of curvature and lipid composition to the formation of lipid-packing defects. ( a ) Packing defect size constants in the outer leaflet of DMPC (blue), POPC (black) and DOPC (magenta) lipid bilayers as a function of total curvature. Linear regression fits are also shown. ( b ) Outer leaflet packing defect size constants in POPC (black), POPC/POG (molar ratio: 85:15, light grey) and POPC/DPPC (molar ratio: 85:15, cyan) bilayers as a function of total curvature. Linear regression fits are also shown. ( c , d ) Curvature-dependent membrane partitioning of ALPS1-ALPS2 in the presence of liposomes of the same compositions as those simulated in a , b . Error bars in a , b indicate s.e. of regression coefficient estimated during the fitting procedure. Vertical error bars in c , d indicate the variation in the relative fluorescence intensity at 530 nm (normalized with respect to the fluorescence of the soluble protein) in two (DMPC, DOPC, POPC/DPPC) or three (POPC, POPC/POG) independent experiments. The horizontal error bars indicate the variation in liposome radius as assessed by dynamic light scattering. Full size image The response of lipid-packing defects to curvature is very similar between POPC and DOPC, while in DMPC the formation of large-packing defects remains scarce even at very high curvatures ( Fig. 4a ). Although the three lipids equilibrate slightly differently between the inner and outer leaflets ( Supplementary Table 1 and Supplementary Fig. 7 ), this mechanism does not appear to counter the intrinsic differences in packing properties that these different lipids display in flat bilayers. Instead, acyl chain unsaturation and curvature have cumulative effects for the formation of lipid-packing defects in these single component lipid bilayers. Of note, acyl chain unsaturation appears as important as curvature for modulating lipid-packing defects. Thus, bending a POPC or a DOPC membrane increases the defect size constant by up to 50%, whereas substituting DOPC for DMPC increases the defect size constant by 30% to 70% depending on the curvature considered. Next, we assessed the membrane interfacial properties when different lipids are added to a POPC matrix. We first prepared mixed POPC/POG and POPC/dipalmitoyl-phosphatidylcholine (DPPC) bilayers with a molar ratio of 85:15 in both inner and outer leaflets, and compared them with pure POPC flat and curved bilayers. POG and DPPC (which is analogous to DMPC but with longer acyl chains to better match the hydrophobic thickness of the POPC bilayers) were chosen because of their opposing shapes. POG is more conical than POPC ( Fig. 2a ) and is expected to promote lipid-packing defects in POPC bilayers, whereas DPPC has a cylindrical shape due to the saturation of its acyl chains and is expected to prevent the formation of lipid-packing defects. These predictions were verified at all curvatures ( Fig. 4b ): POG promotes whereas DPPC prevents the formation of lipid-packing defects in comparison with pure POPC bilayers. To validate the results of these simulations and to further assess the predictive power of the defect size constant, we assessed the partitioning of ArfGAP1 ALPS1-ALPS2 motif on liposomes of the same mixed lipid compositions. In agreement with the simulations, the binding of ALPS1-ALPS2 was extremely sensitive to both membrane composition and curvature ( Fig. 4c ), showing (i) no binding to DMPC vesicles except at very small radii, (ii) high curvature-dependent binding to POPC vesicles and (iii) significant binding to DOPC vesicles even at large radii ( Fig. 4c ). Other ALPS motifs showed qualitatively the same dual sensitivity to membrane curvature and to the acyl chain composition of PC ( Supplementary Fig. 4 ). The results shown in Fig. 4d also confirm the theoretical predictions for two-component bilayers: conical lipids promote, whereas cylindrical lipids decrease, membrane binding with respect to pure POPC bilayers at all curvatures below saturating values. The in vitro data also allow appreciating the predictive power of the CG simulations. The observation that ALPS1-ALPS2 hardly senses the curvature of pure DMPC membranes is consistent with the in silico prediction that the corresponding defect size constant remains below the 11.0 Å 2 threshold value even at the highest curvature. In contrast, ALPS1-ALPS2 senses the curvature of POPC or DOPC bilayers because, in these cases, the defect size constant varies above the 11.0 Å 2 threshold value ( Figs 2d and 4a ). Finally, the ALPS1-ALPS2 peptide binds more favourably to large ( J =0.02 nm −1 , equivalent to R =100 nm) DOPC than to very small ( J =0.1 nm −1 , equivalent to R =20 nm) DMPC vesicles. The corresponding values of the packing defect size constants extrapolated from the linear fits in Fig. 3a are 12.6 and of 9.9 Å 2 , respectively, and thus in perfect agreement with the binding assays. In contrast, we noticed that another area parameter derived from the simulations ( Supplementary Table 1 ), the area per lipid, did not correlate with the partitioning of ALPS1-ALPS2, further highlighting the relevance of lipid-packing defects as an index of the propensity of a given membrane to promote hydrophobic insertions. In conclusion, both experiments and simulations converge to a similar conclusion: membrane curvature and lipid composition synergize rather than oppose each other for the formation of lipid-packing defects and, consequently, for the adsorption of proteins through hydrophobic insertions. Membrane shape has recently emerged as an important regulatory mechanism for the targeting of peripheral proteins, and numerous proteins and peptides have been found to be sensitive to membrane curvature [14] , [35] , [42] , [43] . In addition, it is well established that lipid composition is a key parameter to tune the partitioning of proteins and peptides to lipid bilayers [2] , [4] . However, these two parameters are often conceptually separated when interpreting in vitro experiments even though they combine in cellular contexts. Indeed, membrane curvature is everywhere, but some curvature sensors appear adapted to different environments, for example, taking advantages of either high electrostatics at the PM or loose lipid packing at the ER [4] , [42] , [44] . Using chemical-specific CG MD of lipid bilayers [31] and new methods for membrane surface analysis [25] , [26] , we have shown that the relative contribution of membrane curvature and composition on the interfacial properties of model membranes can be explicitly quantified in silico . Even though current CG force fields have some limitations [45] , here they appear to provide a reliable method to visualize and quantify membrane properties that are otherwise extremely difficult to obtain with structural methods. Moreover, in vitro binding assays demonstrate that the computed properties correlate remarkably well with the membrane adhesive properties of model peptides of the ALPS motif family. As this motif is generic [14] , the conclusions derived from our studies should apply to other proteins that use hydrophobic insertions. A single parameter, the defect size constant, appears to describe quantitatively the ‘surface texture’ of a bilayer, that is, to capture in a single numerical value the combined effect of membrane curvature and lipid composition on the packing arrangement of lipids. Notably, the defect size constant better rationalizes the influence of membrane properties on protein adsorption as compared with more traditional parameters. For instance, the area per lipid increases with positive curvature and with the number of unsaturated acyl chains but decreases on the insertion of conical-shaped lipids ( Supplementary Table 1 ). Consequently, this metrics fails to predict the interplay between membrane composition and curvature on protein adsorption. As an example, the area per lipid is larger in highly curved DMPC vesicles than in flat DOPC bilayers (75 and 65 Å 2 , respectively; see Supplementary Table 1 ); yet, ALPS motifs bind preferentially to the latter membrane. In contrast, the defect size constant is smaller in highly curved DMPC vesicles than in flat DOPC bilayer (9.9 and 11.4 Å 2 , respectively). In continuum models of lipid membranes, changes in membrane curvature or insertion of non-cylindrical lipids are associated with the generation of stresses in the membrane. A recent computational study shows that the membrane-binding coefficient of ALPS motif correlates very well with the interfacial membrane stress [37] . Therefore, lipid-packing defects can be viewed as a molecular description of interfacial membrane stresses used in continuum membrane physics. However, the advantage of describing and quantifying the contributions of lipid shape and membrane curvature at an atomic scale is to better acknowledge the complexity and variety of lipid membrane interfaces [46] . In this study we have focused our analysis on defects extending 1 Å below the glycerol level, as suggested by the observation that ALPS motifs insert bulky hydrophobic residues into such defects [15] . Other membrane-binding proteins as well as amphiphilic compounds used in chemical biology might prefer deeper or shallower defects, depending on the amino acid composition of their hydrophobic moiety [35] , [44] , [47] , [48] . These variations, which are also critical in membrane curvature generation mechanisms [49] , are ignored in models where membrane curvature is assumed to simply increase the number of ‘binding sites’ for peripheral proteins, regardless of the type of hydrophobic moieties [16] , [17] . Therefore, our atomistic approach should be instrumental to better characterize various modes of protein adsorption on membrane organelles. The main limitation of rationalizing protein adsorption through a protein-independent membrane property is that protein-induced membrane deformations are neglected. This approximation should be valid for proteins that work at low surface concentration and sense but do not alter membrane properties. This is especially true for ALPS motifs, which have been shown to not affect the distribution of lipid-packing defects on binding [15] . In fact, the remarkable agreement between protein adsorption and lipid-packing defects observed in this study is a confirmation of the exquisite role of ALPS motifs as sensors of membrane physical properties. However, for amphipathic motifs that actively remodel membranes, the agreement between membrane partitioning and lipid-packing defects might be more limited, as other interactions (such as electrostatics and crowding) are likely to contribute significantly to the overall binding free energy. Our simulations and experiments suggest that the range of packing defect conditions that can be obtained is remarkably large because lipid composition and curvature have, under most conditions, cumulative effects. This is obvious in simulations with a single lipid species (for example, DOPC versus POPC; Fig. 3 ). However, the cumulative effect persists when two lipids with different shape are free to distribute between the outer and inner membrane leaflets ( Supplementary Fig. 8 ). Indeed, in agreement with previous experimental and theoretical studies [19] , [20] , [21] , [22] , [23] , [24] , lipid sorting by membrane shape is not efficient when physiological radii are considered and does not correct significantly lipid-packing defects. Our results have important implications in a cellular context. First, they suggest that the relative abundance of saturated and unsaturated lipids is crucial to tune the interfacial properties of a lipid bilayer and give a potential molecular explanation for why this ratio is tightly controlled [18] , [32] . A corollary of these results is that liquid-ordered domains, which are enriched in saturated lipids, should be unfavourable for protein hydrophobic insertions, an effect that has been observed experimentally [50] , [51] . Second, the cumulative effect of membrane shape and composition suggests that the topography of organelle membranes is highly diverse. Notably, considering that the saturation of bulk phospholipids increases along the secretory pathway, it is likely to be that the ER and the cis -Golgi are the privileged territories for large lipid-packing defects. In the future, the general approach presented here may be refined in several directions: by changing the threshold value of lipid-packing depth, by combining the analysis with electrostatics, by incorporating more complex lipid species, by studying the membrane partitioning of other proteins and by explicit CG modelling of protein adsorption. Together with continuous progresses in organelle fractionation and lipid analysis [6] , [52] , these efforts should help understand the fine cellular distribution of peripheral proteins and notably those containing membrane curvature sensors. Cell biology Immortal human retinal pigmental epithelial (RPE1) cells were purchased from ATCC (Manassas, VA) and cultured on 100-mm dishes (BD Falcon) in DMEM/F12 containing 10% (v/v) heat-inactivated fetal bovine serum at 37 °C in a humidified 5% CO 2 incubator, and a subculture was carried out every 3–4 days. The RPE1 cells stably expressing EGFP-ArfGAP1(R50K) were selected using G418 (Sigma) and were sorted by FACS. For transient transfections, RPE1 cells (8.0 × 10 4 ) were seeded on a 24-well plate with coverslips, cultured for 2 days, washed with PBS twice and starved for 24 h. The plasmids of catalytically inactive ArfGAP1 and ArfGAP3 labelled with EGFP (EGFP-ArfGAP1(R50K) and EGFP-ArfGAP3(R53K), respectively) were transfected using Lipofectamine2000 (Invitrogen) according to the manufacturer’s protocol. Three hours after transfection, the cells were washed with serum-free medium twice and incubated with BSA-conjugated fatty acid (125 μM C16:0 or 125 μM C18:1 in complex with 25 μM BSA) for 3 h. After being washed twice in PBS, the cells were fixed with 3% paraformaldehyde and imaged using a confocal microscope (SP5, Leica) equipped with a × 63 lens (HCX, Plan Apo, oil immersion, numerical aperture 1.40). Z -stack images of fixed cells were acquired every 0.3 μm and were analysed using Volocity (PerkinElmer) and ImageJ (NIH). From the Z -stack projection, we selected three 2 μm × 2 μm regions of interest: at the Golgi apparatus, in the cytosol near the Golgi and outside the cell (background), and the fluorescence level of these three regions was determined. The Golgi/cytosol ratio is given by: ( I Golgi − I background )/( I cytosol − I background ). The fluorescent intensities of Golgi and cytosol regions were quantified to calculate the Golgi/cytosol ratio of each construct. For quantitative analysis of the incorporation of exogenously added fatty acids in cellular phospholipids, RPE1 cells (6.0 × 10 5 ) were seeded on 100-mm dish and cultured for 3 days. The cells were starved for 24 h and then treated with BSA-conjugated fatty acids for 3 h. The cells were washed with PBS twice and were collected using cell scrapers. The cell pellets were obtained by centrifugation (1,000 g , 5 min). Lipids were extracted from the cell pellet and phospholipids were separated from apolar lipids by thin layer chromatography. The phospholipid fraction was then transesterified and the resulting fatty acids were analysed by gas chromatography on a BPX70 column. Lipid analysis was performed by the lipodomics facility of the Institut National des Sciences Appliquées, Lyon. For live-cell imaging, RPE1 cells (1.5 × 10 5 ) stably expressing EGFP-ArfGAP1(R50K) were seeded on a coverslip in six-well plate (BD Falcon) and incubated for 2 days, followed by serum starvation for 24 h. For observation, the cells were treated sequentially with C16:0 (125 μM) for 3 h and with C18:1 (125 μM) for 3 h at 37 °C in a CO 2 incubator. At various stages of the fatty acid treatments, the cells were observed using a spinning disk microscope (PerkinElmer) equipped with a × 60 objective lens (Plan Apo, oil immersion, numerical aperture 1.40). Z -stack images were acquired every 0.3 μm. Image analysis and quantification was performed using Volocity and ImageJ as described above. Molecular dynamics simulations All MD simulations have been performed using the software GROMACS 4 (ref. 53 ). In AA simulations, data sets for pure DMPC, POPC and DOPC, as well as for mixed DOPC/DOG have been used from a previous study [26] , while new data sets for POPC/POG, POPC/POPE and DOPC/DOPE have been obtained using an identical procedure. The Berger model [54] , in combination with the half-ε double-pairlist OPLS method [55] , was used for all lipids, and parameters for POG were obtained from a previous model for DOG [56] , while the TIP3P model [57] was used for water molecules. In all simulations the temperature was kept constant at 300 K using a velocity-rescaling thermostat [58] and the pressure was set at 1 bar using the Parrinello–Rahman barostat [59] . Pressure coupling was applied semi-isotropically and periodic boundaries were applied in all directions. A time step of 2 fs was used and bond lengths were constrained using the LINCS algorithm [60] . The smooth particle-mesh Ewald method [61] was used for evaluating electrostatic interactions, with a real space cut-off of 1.0 nm, a grid of 0.12 nm and an interpolation order of 4. The cut-off for Lennard–Jones interactions was set at 1.0 nm. All coarse-grain simulations are based on the MARTINI force field [31] . The force field for POG and DOG lipids was developed following the basic MARTINI strategy [31] by replacing the two beads corresponding to the choline and the phosphate groups in PC lipids with a single intermediate polar bead ‘Nda’ typical of chemical groups that can act both as hydrogen bond donor and acceptor, as it is the case for the hydroxyl group of diacyl-glycerol. Bond and angle force constants for the new bead were kept identical to the substituted phosphate bead. Non-bonded interactions (electrostatics and Lennard–Jones) were treated using shifted potentials with a cut-off radius of 1.2 nm. Pressure and temperature were controlled through the coupling to an external bath using the Berendsen algorithm [62] , temperature was kept at 300 K in all systems and pressure control was semi-isotropic for flat bilayers and isotropic for vesicular and tubular structures. In all CG systems, a time step of 30 fs was used and a standard time conversion factor of 4 (ref. 31 ) was used to estimate the length of all production and equilibration runs. Vesicles were simulated using mean-field force approximation boundary potentials to replace the bulk solvent not in direct contact with the lipid bilayers [39] , as this method was shown to be able to enhance the formation and equilibration of vesicles, and to accurately reproduce vesicle properties computed using cubic periodic boundary conditions [39] . Single-lipid component vesicles of radii ranging from 15 to 28 nm were self-assembled from a random mixture of lipids and water molecules using the same protocol described in ref. 39 , with a pure spherical layer of water surrounding the random mixture and by applying a purely repulsive potential to the lipid beads. After vesicle formation, lipids were allowed to equilibrate between the two (inner and outer) leaflets, thanks to cylindrical-shaped boundaries (pores) of radius 1.8 nm acting on the acyl chains of the lipids as described in ref. 39 . The vesicles were deemed equilibrated when the lipid ratio between the inner and outer leaflet converged. Production runs were started after an additional equilibration step of 200 ns following the spontaneous sealing of the pores after removal of the additional cylindrical shape boundaries. Single-lipid component tubules were simulated using cubic periodic boundary conditions after spontaneous self-assembly using the following procedure: from pre-equilibrated vesicles, a radial 5-nm-thick slice composed of lipids and water molecules was extracted. The same slice was replicated five times, and the five replicas were juxtaposed at a fixed distance (3 nm between consecutive slices) and water molecules were added to fill the internal and external spaces in the cubic box. During unrestrained MD, tubules spontaneously self-assembled and large pores formed on their surface. The pores sealed on time scales ranging from 150 to 1 μs, with lipid and water molecules equilibrating between inner and outer compartments before the spontaneous sealing of the pores. Production runs were performed after further (2 μs) equilibration of the sealed tubules. Two component (POPC/DPPC and POPC/POG) vesicles and tubules were generated starting from the corresponding POPC vesicles and tubules after (i) removal of the choline bead and replacement of the phosphate bead with the ‘Nda’ bead in the case of POG and (ii) removal of the terminal carbon bead of the oleoyl acyl chain and replacement of the unsaturated central carbon bead with an saturated bead in the oleoyl acyl chain of POPC in the case of DPPC. An identical percentage of lipids (15%) was substituted in the inner and outer leaflets. The mixed bilayers were then minimized and shortly equilibrated (200 ns) before the production runs. Equilibration between inner and outer leaflet in the R =15 vesicles was achieved through cylindrical-shaped boundaries of R =1.8 nm analogously to the procedure described above for single-component vesicles. The following two different starting lipid concentrations, both at 85:15 molar ratio were chosen: (i) an identical percentage of lipids were substituted in both inner and outer bilayer, and (ii) an identical number of lipids were substituted in both the inner and outer bilayer. In all vesicular and tubular structures, the radii were calculated according to the coordinates of NC3 beads. The curvature values discussed in the text refer to the radii computed from the position of outer leaflet lipids only. Additional details (total membrane surface, number of lipids and simulation lengths) for each system are presented in Supplementary Table 1 . All molecular images were rendered with VMD [63] and PyMol [64] . Packing defects analysis In flat membranes, packing defects were computed using the Cartesian method described in ref. 26 . First, in each bilayer leaflet the plane perpendicular to the membrane normal was mapped into a grid of 0.1 nm resolution. At each grid point, the normal to the membrane plane was scanned starting from the solvent and descending up to 1 Å below the nearest glycerol (sn-2 carbon for AA and the deepest bead among GL1 or GL2 for CG simulations, respectively). At each z -position of a given grid point, the presence of a possible overlapping atom was evaluated by calculating the distance between the grid point centre and the centre of any atom of the bilayer. Overlap was assigned when this distance was shorter than the grid point diagonal half-length (0.07 nm) plus the VdW radius of the atom. If no atomic density was met, the grid point was defined as a defect point. Adjacent defect points were then merged, resulting in defects of various sizes. The VdW radii for the AA simulations are identical to those described in ref. 26 , while for CG simulations the VdW radii correspond to 2 1/6 s ij /2, where s ij are the Lennard–Jones parameters for non-bonded interactions with the most apolar types in the MARTINI force field, a choice that was motivated by the observation that ALPS motifs partition into model membranes by inserting bulky hydrophobic residues [15] . The effective VdW radii are thus of 0.264 nm for all CG beads, with the exception of choline and phosphate beads, which have an effective radius of 0.348 nm. For vesicular and tubular structures, the algorithm was converted into spherical and cylindrical coordinates, respectively, and lipid-packing defects were identified by scanning along the radial direction. To define the grid for the scanning procedure, the membrane was divided into patches of sizes containing between 150 and 500 lipids, and the average radius of glycerol atoms in the patch was selected as the reference point ( R gly ). Grid points were subsequently selected by dividing the geodetic at R gly into segments of length 0.1 nm. Scanning along the radial coordinate was then performed at each grid point by descending up to 0.1 nm below the nearest glycerol, in analogy with the procedure on flat bilayers. Using this discretization procedure, the grid length (and hence the method resolution) was always in the 0.095 to 0.105 nm range. Defects were computed every 100 ps for AA trajectories and every 300 ps for CG trajectories. The histograms of the computed packing defects versus defect size, normalized with respect to the total surface area analysed, were then fitted with a single-exponential distribution y = A *exp(− x / x 0 ) for x >20 Å 2 . The resulting x 0 values are the packing defect size constants used throughout the text. Error bars shown in the text are s.e. in x 0 values estimated during the fitting procedure. Peptide purification and NBD labelling The NBD labelled peptides were prepared as previously described [27] . Briefly, the ALPS1 and ALPS1-ALPS2 peptides (residues 192–257 and 192–304 of ArfGAP1, respectively) carrying the A236C mutation were expressed in Escherichia coli as glutathione S-transferase (GST) fusions. The transformed bacteria were resuspended in 50 mM Tris (pH 7.4) and 150 mM NaCl (TN buffer) supplemented with 1 mM dithiothreitol (DTT), 1 mM phenylmethylsulphonyl fluoride, 1 μM pepstatin, 10 μM bestatin, 10 μM phosphoramidon and a cocktail of anti-proteases (Roche). The lysate was prepared using a French press. The supernatant was incubated for 2 h with glutathione-Sepharose 4B beads (Amersham). The beads were washed three times with TN buffer containing 1 mM DTT and were incubated with thrombin at 4 °C overnight, followed by the elution of the peptide. The peptide was purified by HPLC using a Chromolith C18 column (Merck) with an acetonitrile gradient. The ALPS GMAP peptide (GMAP210 residues 1–38) carrying the M1C mutation was purchased from ProteoGenix. For NBD labelling, the peptides were resuspended in 50 mM HEPES (pH 7.2) and 120 mM potassium acetate (HK buffer), and labelled with NBD on the cysteine residue. The labelled peptides were purified by HPLC. The peptide concentration and the extent of NBD labelling (≈1 mol:mol) were determined from the absorbance at 280 and 500 nm. Liposome preparation POPC, POPE, POG, DPPC, DOPC, DOPE, DOG and DMPC in chloroform were purchased from Avanti Polar Lipids. Lipid films of POPC, POPC/POPE (85/15 mol%), POPC/POG (85/15), POPC/DPPC (85/15), DOPC, DOPC/DOPE (85/15), DOPC/DOG (85/15) and DMPC were prepared by evaporation. The films were resuspended in HK buffer containing 2 mM DTT to reach a lipid concentration of 2 mM. After five freezing/thawing cycle in liquid nitrogen, the lipid suspensions were sequentially extruded using a hand extruder (Avanti). Large (≈flat) liposomes were prepared by extrusion through 0.4 μm filters. Liposomes of decreasing size were prepared by sequentially extrusion through 0.2, 0.1, 0.05 and 0.03 μm pore-size polycarbonate filters. Very small liposomes were prepared by sonication using a titanium tip (Misonix). Titanium and lipid debris were removed by centrifugation at 100,000 g for 20 min. Liposome radius was estimated by dynamic light scattering using a Dyna Pro instrument. Liposomes were stored at room temperature and used within 1 day. NBD fluorescence measurements of ALPS partitioning Emission fluorescence spectra from 520 to 680 nm (bandwidth of 5 nm) were recorded on excitation at 505 nm (bandwidth of 5 nm) in a 100-μl quartz cuvette using a Shimadzu R-5301-PC spectrofluorometer for the following mixtures: (i) HK buffer supplemented with 1 mM MgCl 2 (HKM buffer) (ii) liposomes (300 μM) of defined radius in HKM buffer and (iii) each NBD-labelled peptide (final conc. 0.25 μM) in combination with either HKM buffer or liposome buffer after mixing by pipetting. The corrected emission spectra of the NBD-labelled peptides were then obtained by subtracting the emission spectra without peptide to remove light scattering and background signals. The fluorescence intensity ( F ) at 530 nm of the NBD-labelled peptide in each condition was then normalized by setting the fluorescence intensity ( F 0 ) of the peptide in HKM buffer to an arbitrary value of 1. The relative fluorescence intensity ( F / F 0 ) at 530 nm was plotted as a function of total curvature (in nm −1 ) or lipid concentration. In the later case, data were fit according to the quadratic equation [27] : where [L t ] and [P t ] are the total lipid and peptide concentration, n the number of lipids occupied by the bound peptide and K the apparent equilibrium constant between the peptide and the lipid patch of n lipids, The partitioning coefficient (in M) is given by Kp = nK . Statistics For lipidomics, Bonferroni test after analysis of variance was carried out to compare the acyl chain content of phospholipids from three groups (without fatty acids, C16:0 and C18:1) pooled from four independent experiments. For the Golgi/cytosol ratio of ArfGAP proteins, Kruskal–Wallis test and two-tailed Mann–Whitney U -test with Bonferroni correction were performed to compare three groups (without fatty acids, C16:0 and C18:1) pooled from three independent experiments. How to cite this article: Vanni, S. et al. A sub-nanometre view of how membrane curvature and composition modulate lipid packing and protein recruitment. Nat. Commun. 5:4916 doi: 10.1038/ncomms5916 (2014).